A fluorinated dendrimer achieves excellent gene transfection efficacy at extremely low nitrogen to phosphorus ratios Polymers have shown great promise in the design of high efficient and low cytotoxic gene vectors. Here we synthesize fluorinated dendrimers for use as gene vectors. Fluorinated dendrimers achieve excellent gene transfection efficacy in several cell lines (higher than 90% in HEK293 and HeLa cells) at extremely low N/P ratios. These polymers show superior efficacy and biocompatibility compared with several commercial transfection reagents such as Lipofectamine 2000 and SuperFect. Fluorination enhances the cellular uptake of the dendrimer/DNA polyplexes and facilitates their endosomal escape. In addition, the fluorinated dendrimer shows excellent serum resistance and exhibits high gene transfection efficacy even in medium containing 50% FBS. The results suggest that fluorinated dendrimers are a new class of highly efficient gene vectors and fluorination is a promising strategy to design gene vectors without involving sophisticated syntheses. Cationic polymers are widely used as promising gene vectors to introduce exogenous nucleic acid into cells [1] , [2] , [3] , [4] , [5] , [6] , [7] . These materials are easy-to-manufacture and have superior safety compared with viral gene vectors; however, their commercial and clinical applications are limited by relatively low transfection efficacy and poor cell viability after transfection [8] , [9] , [10] , [11] . Functionalization of polymers with amino acids [12] , lipids [13] , cyclodextrins [14] , peptides [15] , other polymers [16] and inorganic nanoparticles [17] can improve their transfection efficacy and biocompatibility to some extent, but the resulting materials are still not efficient enough to justify clinical uses. Fluorine is absent in biological systems, but is widely used to tailor the properties or behaviours of drugs, biomacromolecules and cells [18] , [19] , [20] , [21] , [22] . Fluorination increases the therapeutic efficacy or pharmacokinetic behaviour of numerous drugs [18] , [19] , improves the stability of proteins without altering their structures and functions [21] , and allows the detection or imaging of the labelled compounds using magnetic resonance imaging or positron emission tomography imaging [23] , [24] . Fluorinated compounds are both hydrophobic and lipophobic, and have a high phase-separation tendency in both polar and non-polar environments [25] , [26] . Therefore, fluorination can improve the affinity of polymers to cell membrane [27] and across the lipid bilayer of the cell membrane, as well as the endosome/lysosome membrane [28] , facilitating endosomal escape of the polymers. In addition, fluorinated polymers have low surface energy and prefer to associate with each other at low concentrations [29] , [30] , [31] , allowing the formation of polyplexes with nucleic acid at low nitrogen to phosphorus (N/P) ratios. Gene transfection at a low N/P ratio is essential to minimize the toxicity on the transfected cells. Dendrimers with versatile properties are frequently used in the field of biomaterials and nanomedicine [32] , [33] , [34] , [35] , [36] , [37] . These polymers are monodisperse and can be easily modified with fluorous compounds [38] , [39] . Here we propose a fluorination strategy to dramatically improve the efficacy of cationic polymers while reducing their cytotoxicity in gene transfection. We synthesize fluorinated dendrimers by a facile route and use them as a new class of polymeric gene vectors. The fluorinated dendrimers fulfill the two main requirements in gene delivery—dramatic transfection efficacy and low cytotoxicity. Fluorination also works well on other cationic polymers such as poly(ethylenimine) in gene delivery and represents a promising tool in the design of high efficient and low cytotoxic gene materials. Characterization of fluorinated dendrimers Generation 5 (G5) poly(amidoamine) (PAMAM) dendrimers were reacted with perfluoro acid anhydrides at room temperature to yield fluorinated dendrimers ( Fig. 1a ). 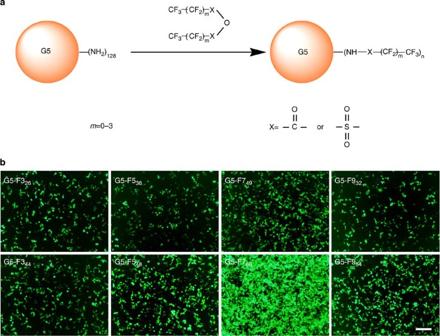Figure 1: Synthesis and gene transfection efficacy of fluorinated dendrimers. (a) Synthetic route of the fluorinated dendrimers. (b) EGFP gene transfection efficacies of the synthesized fluorinated dendrimers in HEK293 cells at their optimized N/P ratios listed inSupplementary Fig. 1. Scale bar, 200 μm. The number of perfluoro acid modified on each G5 dendrimer is evaluated by a well-established ninhydrin assay ( Supplementary Table 1 ). The resulting materials are termed G5-F3 26 , G5-F3 44 , G5-F5 36 , G5-F5 48 , G5-F7 49 , G5-F7 68 , G5-F9 32 and G5-F9 54 , respectively. Gene transfection efficacy of these fluorinated dendrimers at their optimized N/P ratios were tested in HEK293 cells using an enhanced green fluorescent protein (EGFP) plasmid. As shown in Fig. 1b and Supplementary Fig. 1 , heptafluorobutyric acid-modified dendrimers (G5-F7 68 and G5-F7 49 ) show much higher transfection efficacy in HEK293 cells than other fluorinated dendrimers. Therefore, G5-F7 68 and G5-F7 49 were investigated in detail in further gene transfection studies. Figure 1: Synthesis and gene transfection efficacy of fluorinated dendrimers. ( a ) Synthetic route of the fluorinated dendrimers. ( b ) EGFP gene transfection efficacies of the synthesized fluorinated dendrimers in HEK293 cells at their optimized N/P ratios listed in Supplementary Fig. 1 . Scale bar, 200 μm. Full size image Fluorination improves transfection efficacy of dendrimers As expected, both G5-F7 68 and G5-F7 49 effectively form polyplexes with DNA ( Supplementary Fig. 2 ) and condense the plasmid DNA into 100–200 nm nanoparticles even at an extremely low N/P ratio of 0.5 ( Supplementary Figs 3 and 4 ). Vierling et al. [40] increased the transfection efficacy of cationic lipids through fluorination. However, the fluorinated cationic lipids must be typically co-formulated with non-fluorinated lipids and only show moderate increases in transfection efficacy [40] , [41] . Here, fluorination significantly improves the EGFP transfection efficacy of a G5 dendrimer (from 21.8 to 69.9% for G5-F7 49 and 97.1% for G5-F7 68 ) in HEK293 cells ( Fig. 2a,b ). High efficacy of G5-F7 68 achieves at an extremely low N/P ratio of 1.5, and its efficacy is higher than Lipofectamine 2000 (70.8%), a commercial transfection reagent. Similar results were obtained using a luciferase reporter gene ( Fig. 2c ). The high transfection efficacy of G5-F7 68 is further confirmed in HeLa cells ( Fig. 3 and Supplementary Fig. 5 ), COS-7 cells ( Supplementary Fig. 6 ), CHO cells ( Supplementary Fig. 7 ) and NIH3T3 cells ( Supplementary Fig. 8 ). G5-F7 68 shows higher efficacies than Lipofectamine 2000 in most of the cells, except in CHO cells ( Fig. 4 ). G5-F7 68 is also more efficient than SuperFect, branched poly(ethylenimine) with a molecular weight of 25 kDa (bPEI25K), lysine- and arginine-modified G5 dendrimers (G5-Lys 130 and G5-Arg 108 ), which were shown to be effective in introducing DNA into cells such as HeLa cells ( Fig. 4b ) [42] . Even at an extremely low N/P ratio of 0.5, relatively high EGFP gene expressions (~50%) in HeLa and HEK293 cells were observed for the G5-F7 68 /DNA polyplexes ( Supplementary Fig. 9 and Supplementary Note 1 ). Gene transfection at a low N/P ratio ensures low cytotoxicity of the materials during gene transfection [43] . As shown in Fig. 4a and Supplementary Fig. 10 , G5-F7 68 and G5-F7 49 show low cytotoxicity (>90% cell viability) on these cells. In addition, G5-F7 68 shows reproducible gene transfection in HeLa cells ( Supplementary Fig. 11 ). These results suggest that G5-F7 68 is an efficient and biocompatible vector for the introduction of both EGFP and luciferase genes into a list of commonly used cells. 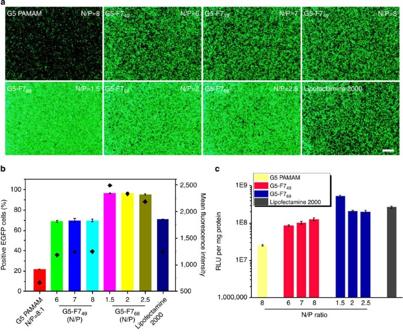Figure 2: Transfection efficacies of fluorinated dendrimers in HEK293 cells. Comparison of fluorinated dendrimers (G5-F749and G5-F768) with G5 and Lipofectamine 2000 on thein vitroEGFP (a,b) and luciferase (c) gene transfection efficacy in HEK293 cells after 24 h. Positive EGFP cells (%) were determined by flow cytometry (b) and the luciferase gene expression level (c) is expressed as relative luciferase light units per milligram of protein (RLU per mg protein). Error bars inbandcrepresent the s.e. (n=3). Diamonds inbrepresent mean fluorescence intensity. Scale bar, 400 μm. Figure 2: Transfection efficacies of fluorinated dendrimers in HEK293 cells. Comparison of fluorinated dendrimers (G5-F7 49 and G5-F7 68 ) with G5 and Lipofectamine 2000 on the in vitro EGFP ( a , b ) and luciferase ( c ) gene transfection efficacy in HEK293 cells after 24 h. Positive EGFP cells (%) were determined by flow cytometry ( b ) and the luciferase gene expression level ( c ) is expressed as relative luciferase light units per milligram of protein (RLU per mg protein). Error bars in b and c represent the s.e. ( n =3). Diamonds in b represent mean fluorescence intensity. Scale bar, 400 μm. 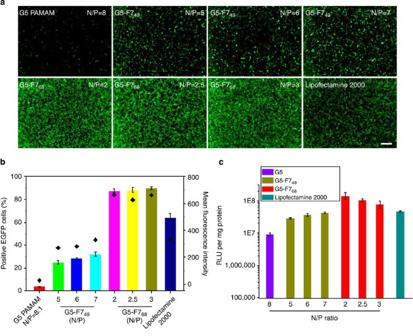Figure 3: Transfection efficacies of fluorinated dendrimers in HeLa cells. Comparison of fluorinated dendrimers with G5 and Lipofectamine 2000 on thein vitroEGFP (a,b) and luciferase (c) gene transfection efficacy in HeLa cells after 48 h. Error bars inbandcrepresent the s.e. (n=3). Diamonds inbrepresent mean fluorescence intensity. Scale bar, 400 μm. Full size image Figure 3: Transfection efficacies of fluorinated dendrimers in HeLa cells. Comparison of fluorinated dendrimers with G5 and Lipofectamine 2000 on the in vitro EGFP ( a , b ) and luciferase ( c ) gene transfection efficacy in HeLa cells after 48 h. Error bars in b and c represent the s.e. ( n =3). Diamonds in b represent mean fluorescence intensity. Scale bar, 400 μm. 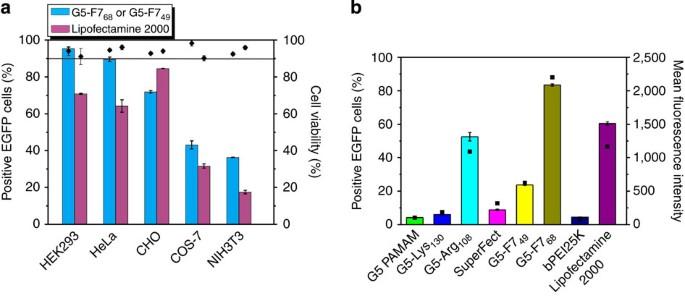Figure 4: Comparison of fluorinated dendrimers with other transfection reagents on gene transfection efficacy. EGFP expression and cell viability in five cell lines transfected by fluorinated dendrimers and Lipofectamine 2000 (a). Diamonds inarepresent cell viability (%). Comparison of fluorinated dendrimers with G5 PAMAM, G5-Lys130, G5-Arg108, SuperFect, bPEI25K and Lipofectamine 2000 on EGFP transfection efficacy at their optimized condition in HeLa cells after 48 h (b). Squares inbrepresent mean fluorescence intensity. Full size image Figure 4: Comparison of fluorinated dendrimers with other transfection reagents on gene transfection efficacy. EGFP expression and cell viability in five cell lines transfected by fluorinated dendrimers and Lipofectamine 2000 ( a ). Diamonds in a represent cell viability (%). Comparison of fluorinated dendrimers with G5 PAMAM, G5-Lys 130 , G5-Arg 108 , SuperFect, bPEI25K and Lipofectamine 2000 on EGFP transfection efficacy at their optimized condition in HeLa cells after 48 h ( b ). Squares in b represent mean fluorescence intensity. Full size image Transfection mechanisms of fluorinated dendrimers To verify the role of fluorine on the high transfection efficacy of G5-F7 68 , we synthesized butyric acid-modified G5 dendrimer, termed G5-H7 69 ( Supplementary Fig. 12 ). As shown in Supplementary Fig. 13 , G5-H7 69 shows extremely weak EGFP transfection efficacy on HEK293 and HeLa cells, suggesting that fluorine modified on dendrimer surface plays an essential role in the efficient gene transfection by G5-F7 68 . We also tested the gene transfection efficacy of G5 dendrimer/perfluorobutyric acid physical mixture. As shown in Supplementary Fig. 14 , the addition of perfluorobutyric acid does not enhance the gene transfection efficacy of G5 dendrimer, suggesting that perfluorobutyric acid should be covalently attached to dendrimer surface to yield an efficient gene vector, such as G5-F7 68 . To investigate the reason behind the high transfection efficacy of fluorinated dendrimers, we compared the cellular uptake and endosomal escape behaviours of G5/DNA and fluorinated G5/DNA polyplexes. As shown in Fig. 5a , fluorination significantly improves the cellular uptake efficacy of DNA bound on G5 dendrimer. G5-F7 68 shows the highest efficacy on delivering DNA into HeLa cells. Fluorination also facilitates the endosomal escape of dendrimer/DNA polyplexes. The addition of bafilomycin A1, which inhibits the acidification in endosome and lysosome, can efficiently block the transfection of EGFP gene by G5-F7 68 , whereas the supplement of sucrose, a lysosomotropic agent that accelerates the escape of polyplexes from acidic vesicles, cannot further improve the transfection efficacy of G5-F7 68 ( Supplementary Fig. 15 ) [44] , [45] . The efficient cellular uptake and endosomal escape of G5-F7 68 /DNA polyplexes are further confirmed by confocal microscopy. DNA (labelled with a green fluorescent dye, YOYO-1) delivered by G5-F7 68 showed efficient cellular uptake (~100%) in HeLa cells and most of the DNA escaped from the acidic vesicles stained by LysoTracker Red within 4 h ( Fig. 5b ); however, G5/DNA and G5-F7 49 /DNA polyplexes shows less efficient cellular uptake than G5-F7 68 /DNA polyplexes. Co-localizations of YOYO-1 within the acidic vesicles are observed for these polyplexes at 4 h ( Fig. 5b and Supplementary Fig. 16 ). 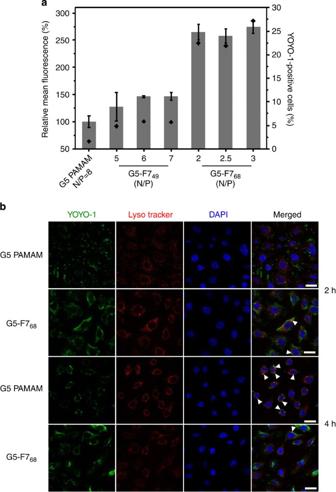Figure 5: Cellular uptake and endosomal escape abilities of fluorinated dendrimers in HeLa cells. (a) Cellular uptake of YOYO-1-labelled DNA delivered by G5, G5-F749and G5-F768, respectively. The samples were incubated with HeLa cells for 1 h. Error bars represent the s.e. (n=3). Diamonds represent YOYO-1-positive cells (%). (b) Confocal images of HeLa cells treated with G5-F768/DNA and G5/DNA polyplexes for 2 and 4 h, respectively. DNA was labelled with YOYO-1, the endosomes were stained with LysoTracker Red and the nuclei were stained with DAPI (4′,6-diamidino-2-phenylindole). The arrows indicate co-localization of YOYO-1-labelled DNA and LysoTracker Red-stained endosomes in HeLa cells. Scale bar, 20 μm. Figure 5: Cellular uptake and endosomal escape abilities of fluorinated dendrimers in HeLa cells. ( a ) Cellular uptake of YOYO-1-labelled DNA delivered by G5, G5-F7 49 and G5-F7 68 , respectively. The samples were incubated with HeLa cells for 1 h. Error bars represent the s.e. ( n =3). Diamonds represent YOYO-1-positive cells (%). ( b ) Confocal images of HeLa cells treated with G5-F7 68 /DNA and G5/DNA polyplexes for 2 and 4 h, respectively. DNA was labelled with YOYO-1, the endosomes were stained with LysoTracker Red and the nuclei were stained with DAPI (4′,6-diamidino-2-phenylindole). The arrows indicate co-localization of YOYO-1-labelled DNA and LysoTracker Red-stained endosomes in HeLa cells. Scale bar, 20 μm. Full size image Fluorinated dendrimer shows excellent serum resistance The gene transfection using fluorinated dendrimers in this study was conducted in medium containing 10% fetal bovine serum (FBS). As shown in Fig. 6 , G5-F7 68 preserves efficient gene transfection (55.4%) in HeLa cells even in medium containing 50% FBS, whereas Lipofectamine 2000 almost lost its transfection efficacy in medium containing 30% FBS. The excellent serum resistance of G5-F7 68 in gene delivery is attributed to the inactive surface of fluorinated dendrimer against serum proteins. This result shows encouraging gene delivery potential of G5-F7 68 for in vivo applications. 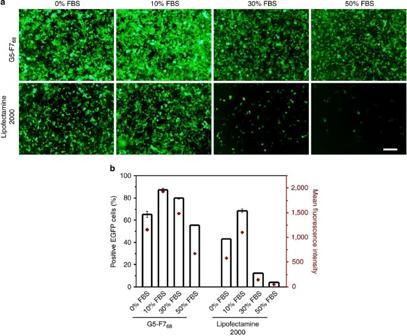Figure 6: Serum-resistance abilities of fluorinated dendrimers on EGFP gene transfection. EGFP expression in HeLa cells were performed using G5-F768(N/P ratio at 2.5:1) and Lipofectamine 2000 in mediums containing 0%, 10%, 30% and 50% FBS, respectively (a). The EGFP gene transfection efficacy was determined by flow cytometry (b). Error bars inbrepresent the s.e. (n=3). Diamonds inbrepresent mean fluorescence intensity. Scale bar, 200 μm. Figure 6: Serum-resistance abilities of fluorinated dendrimers on EGFP gene transfection. EGFP expression in HeLa cells were performed using G5-F7 68 (N/P ratio at 2.5:1) and Lipofectamine 2000 in mediums containing 0%, 10%, 30% and 50% FBS, respectively ( a ). The EGFP gene transfection efficacy was determined by flow cytometry ( b ). Error bars in b represent the s.e. ( n =3). Diamonds in b represent mean fluorescence intensity. Scale bar, 200 μm. Full size image The transfection efficacy of a polymeric gene vector depends on multiple parameters, that is, DNA condensation and protection, serum stability, cellular uptake efficiency, intracellular trafficking such as endosomal escape, DNA unpacking and nuclear entry [8] . As demonstrated above, fluorination on dendrimers enhances cellular uptake, endosomal escape and serum resistance of the dendrimer/DNA polyplexes. It also modulates the DNA packing/unpacking ability of the dendrimers. As shown in Supplementary Fig. 17 , G5-F7 68 is easier to release its bound DNA in the presence of heparin than G5 dendrimer, owing to the low N/P ratio of G5-F7 68 /DNA polyplexes, to the reduced surface charge density on dendrimer surface after fluorination and to the inert surface of fluorinated dendrimer towards the bound DNA. If a plasmid DNA is loosely bound with the vector, it will be rapidly degraded by cytosolic nuclease. On the contrary, tight binding makes it difficult for DNA unpacking and leads to failed gene transfection [8] . Dendrimer is such a material that has strong binding ability with DNA owing to the multivalency effect of the surface charges. The incorporation of an anionic polymer into the dendrimer/DNA polyplex can increase the DNA release rate and improve the transfection efficacy of cationic dendrimers [46] , [47] . Therefore, the easier DNA unpacking ability of G5-F7 68 compared with unmodified dendrimer might be one of the reasons to explain the dramatic efficacy of G5-F7 68 in gene delivery. It is worth noting that perfluoroaliphatic acid is a protecting group for amines and the corresponding amide could be hydrolysed under basic conditions. Surprisingly, the stability of fluorinated dendrimer G5-F7 68 is excellent in aqueous solutions ( Supplementary Fig. 18 ). G5-F7 68 maintains efficient gene transfection after the samples were stored at −20 °C for 8 months ( Supplementary Fig. 11 ). Even if the fluorinated dendrimer is degraded in the cells, it will not induce additional toxicity on the transfected cells. As shown in Supplementary Fig. 19 , both G5-F7 68 and G5/heptafluorobutyric acid mixture (fully degraded products of G5-F7 68 ) are non-toxic on the cells, suggesting the excellent biocompatibility of the fluorinated dendrimer in gene delivery. One may ask why G5-F7 68 has a much higher transfection efficacy than other fluorinated dendrimers. A possible answer is suggested by a balance of several factors influencing the transfection efficacy, such as chain length of the perfluoroaliphatic acid, number of conjugated ligands and residual surface charges, and degradability of the fluorinated dendrimer. This phenomenon is also observed in the gene transfection efficacies of dendrimers modified with aliphatic acid of different chain lengths [48] . The exact reason behind this question needs further investigations on the fluorinated dendrimers. In summary, fluorinated dendrimer G5-F7 68 achieves high gene transfection efficacy even at extremely low N/P ratio around 0.5. The efficacy of G5-F7 68 is higher than several commercial gene reagents such as Lipofectamine 2000 and SuperFect in a list of cells. Low dose of the G5-F7 68 used ensures high viability of the cells during gene transfection. Fluorination removes the association of transfection efficacy and cytotoxicity for dendrimer-based gene delivery systems. The increased transfection efficacy of dendrimer after fluorination is mainly attributed to increased cellular uptake and facilitated endosomal escape of the polyplexes. In addition, G5-F7 68 shows excellent serum resistance and even exhibits high transfection efficacy in medium containing 50% FBS. Not limited to G5 PAMAM dendrimer, fluorination also works well on other dendrimer generations (such as G4 PAMAM dendrimer, Supplementary Fig. 20 ), other dendrimer species (such as polypropylenimine dendrimer, Supplementary Fig. 21 ) and other cationic polymers (such as bPEI25K, Supplementary Fig. 22 ). All these fluorinated materials achieved high transfection efficacies at low N/P ratios. Taken together, G5-F7 68 showed dramatic gene transfection efficacy in commonly used cell lines. Fluorination on polymers as well as other biomaterials can be used as a versatile tool in the development of efficient drug and gene carriers. Further work will be focused on investigating the exact mechanism of fluorination on gene delivery and evaluating the in vivo efficacy of fluorinated polymers such as G5-F7 68 on the delivery of therapeutic DNAs into tumour-bearing mice. Materials Ethylenediamine-cored G5 PAMAM dendrimer was purchased from Dendritech, Inc. (Midland, MI). Trifluoroacetic anhydride, pentafluoropropionic anhydride, heptafluorobutyric anhydride, nonafluorobutanesulphonic anhydride, butyric anhydride, bafilomycin A1 and sucrose were purchased from Sigma-Aldrich (St Louis, MO). The chemicals were used as received without further purification. Synthesis and characterization of fluorinated dendrimers G5 PAMAM dendrimer and perfluoro acid anhydrides were dissolved in methanol at different molar ratios. The mixtures were stirred at room temperature for 48 h and dialysed against PBS buffer and distilled water. The products were lyophilized under vacuum to obtain fluorinated dendrimers as white gels. The number of remaining amine groups on each fluorinated G5 dendrimer was evaluated by a well-established ninhydrin assay ( Supplementary Method ). The numbers of perfluoro acid modified on G5 dendrimers are listed in Supplementary Table 1 . The synthesis of butyric acid-modified G5 dendrimer was conducted using a similar method as described above, and the number of butyric acid modified on each G5 dendrimer was determined using 1 H NMR. Characterization of fluorinated dendrimer/DNA polyplexes Fluorinated dendrimers, including G5-F7 68 and G5-F7 49 , and unmodified G5 were mixed with DNA at different N/P ratios (0:1, 0.5:1, 1:1, 2:1, 4:1 and 8:1) for 30 min. The samples were electrophoresed on 1% agarose gels and stained by ethidium bromide for 1 h. To compare the stability of G5-F7 68 /DNA and G5/DNA, the polyplexes at an N/P ratio of 2:1 or 8:1 in the presence of different concentrations of heparin were also analysed using agarose gel electrophoresis. Size and zeta-potential of the fluorinated dendrimer/DNA polyplexes were further characterized at 25 °C using dynamic light scattering (Zetasizer Nano ZS90, Malvern Zetasizer 3000). Cell culture and gene transfection HEK293 (a human embryonic kidney cell line, ATCC), HeLa (a human cervical carcinoma cell line, ATCC), NIH3T3 (mouse embryo fibroblasts, ATCC), COS-7 (a fibroblast-like cell line derived from monkey kidney, ATCC) and CHO (a Chinese hamster ovary cell line, ATCC) cells were cultured in DMEM (GIBCO) containing penicillin sulphate (100 units ml −1 ), streptomycin (100 μg ml −1 ) and 10% heat-inactived FBS (GIBCO). The cells were cultured in 24-well plates for 24 h before in vitro gene transfection, followed by the incubation of dendrimer/DNA polyplexes (0.8 μg DNA, the polyplexes were prepared at different N/P ratios and dissolved in 250 μl DMEM containing 10% FBS) with the cells for 6 h. Next, 500 μl fresh DMEM containing 10% FBS were added. Commercial transfection reagents such as Lipofectamine 2000 and SuperFect were used as controls, and gene transfection by these materials were conducted according to the product’s protocols (Invitrogen). The optimized N/P ratios for other controls such as unmodified G5 PAMAM dendrimer, bPEI25K, G5-Lys 130 and G5-Arg 108 were screened before their comparisons on transfection efficacy with fluorinated dendrimers. The gene transfection experiments were conducted for 24 h (HEK293 cells) or 48 h (other cell lines). The expression of EGFP plasmid in the cells was directly observed by a fluorescent microscopy (Olympus, Japan), and the transfection efficacy was quantitatively measured using flow cytometry. The determination of luciferase plasmid expression was performed according to the manufacturer’s protocols (Promega). The luciferase activities were normalized with respect to protein concentrations (relative luciferase light units per milligram protein). To investigate the serum resistance of the fluorinated dendrimers, gene transfection experiments for G5-F7 68 and Lipofectamine 2000 were also conducted on HeLa cells in medium containing 0, 10, 30 and 50% FBS. Cellular uptake and gene transfection mechanisms To investigate the cellular uptake efficacies of fluorinated dendrimer/DNA and unmodified dendrimer/DNA polyplexes, DNA was labelled with YOYO-1 (Y3601, Invitrogen) for 10 min before the preparation of polyplexes; HeLa cells were then incubated with the YOYO-1-labelled polyplexes for 1 h and uptake efficacy was analysed using flow cytometry. To investigate the effect of fluorination on the endosomal escape of dendrimer/DNA polyplexes, YOYO-1 was used to monitor intracellular trafficking behaviours of the polyplexes. The cells were incubated with the polyplexes for 2 or 4 h. The acidic vesicles and the nuclei of HeLa cells were then stained with a red fluorescent dye (LysoTracker Red, DND-99, Invitrogen) and a blue fluorescent dye (4′,6-diamidino-2-phenylindole), respectively. Co-localizations of the polyplexes with acidic vesicles in HeLa cells were observed by a laser scanning confocal microscopy (Olympus FV1000). Sucrose and bafilomycin A1 was also used to evaluate the endosome escape abilities of the polyplexes. In general, sucrose (5 mM) and bafilomycin A1 (300 nM) were applied to the cells 1 h before the addition of dendrimer/EGFP plasmid polyplexes. The transfection experiments were conducted as described above. EGFP expressions in HeLa cells treated with and without sucrose or bafilomycin A1 were examined by flow cytometry. The polyplexes for unmodified G5 PAMAM dendrimer and fluorinated dendrimers in the cellular uptake and endosomal escape experiments are prepared at their optimal N/P ratios on HeLa Cells. Cytotoxicity analysis To determine the cytotoxicity of G5-F7 49 and G5-F7 68 , an MTT (3-(4,5-dimethylthiazol-2-yl)-2,5-diphenyltetrazolium bromide) assay was performed in 96-well plates according to well-established protocols. The cells were incubated with fluorinated dendrimers at concentrations equal to that used in gene transfection experiments for 24 h or 48 h. Lipofectamine 2000 and unmodified G5 dendrimer were used as controls. Five repeats were conducted for each sample and the data were given as mean±s.e.m. and analysed by Students’ t -test. How to cite this article: Wang, M. et al. A fluorinated dendrimer achieves excellent gene transfection efficacy at extremely low nitrogen to phosphorus ratios. Nat. Commun. 5:3053 doi: 10.1038/ncomms4053 (2014).